Time-bin entangled photons from a quantum dot Long-distance quantum communication is one of the prime goals in the field of quantum information science. With information encoded in the quantum state of photons, existing telecommunication fibre networks can be effectively used as a transport medium. To achieve this goal, a source of robust entangled single-photon pairs is required. Here we report the realization of a source of time-bin entangled photon pairs utilizing the biexciton–exciton cascade in a III/V self-assembled quantum dot. We analyse the generated photon pairs by an inherently phase-stable interferometry technique, facilitating uninterrupted long integration times. We confirm the entanglement by performing quantum state tomography of the emitted photons, which yields a fidelity of 0.69(3) and a concurrence of 0.41(6) for our realization of time-energy entanglement from a single quantum emitter. A source of entangled photon pairs is essential for quantum communication [1] , [2] and linear optics quantum computing [3] . Quantum information protocols such as quantum teleportation [4] , [5] and entanglement swapping [6] , [7] use entangled photons to enable long-distance distribution of entanglement through quantum repeaters [8] . Optical fibres are the medium of choice for distribution, with the existing extensive global telecommunication fibre network. Polarization entangled photons suffer from decoherence in optical fibres due to polarization mode dispersion [9] , [10] . This effect results in the wavelength and time-dependent splitting of the principal states of polarization with a differential group delay. Thus the arrival time of the photons carries information about their polarization state causing decoherence. Alternatively, time-bin entangled photons [11] are immune to these decoherence mechanisms and are more robust [12] , [13] in optical fibres [12] . At present, spontaneous parametric down-conversion is widely used as a source of time-bin entangled photons [11] . Nevertheless, photons produced by a single quantum emitter show inherently sub-Poissonian statistics [14] . Thus, in this work, we show that the photon cascade in a single semiconductor quantum dot can produce time-bin entangled photon pairs. So far, experimental efforts have been focused on utilizing the biexciton–exciton cascade of a semiconductor quantum dot as a source of polarization entangled photons [15] , [16] , [17] , [18] . A major hurdle in the realization of these sources comes from the asymmetry of the self-assembled quantum dots that results in non-degenerate exciton polarization states, thereby revealing the polarization state of the emitted photons. This hurdle has been overcome by some groups with great effort [19] , [20] , [21] , [22] , [23] , but these technologies are not generally available. Our entanglement scheme combines the strength of a quantum dot as a single-photon source and the robustness of time-bin entanglement. We use only one exciton polarization cascade so that the emitted photons are in a well-defined polarization mode. Nevertheless, our scheme is fairly insensitive to the polarization non-degeneracy; the polarization of the detected photon does not contain any information about the creation time-bin of the photon pair. Schemes to generate single pairs of time-bin entangled photons using the biexciton cascade in a quantum dot have been proposed [24] , [25] . While these schemes require the quantum dot to be initially prepared in a long-living metastable state, we implement time-bin entanglement through resonant excitation of the biexciton from the ground state. This method can produce maximally entangled states but it does not completely suppress double excitations. In this work we show time-bin entanglement generated by a single quantum emitter. Our measurement yields a fidelity of 0.69(3) and a concurrence of 0.41(6). Writing the quantum superposition To excite the quantum dot we use a pump interferometer that transforms the incoming laser pulse into a coherent superposition of two pulses that form well-defined time bins ‘early’ and ‘late’. The delay in the pump interferometer is set such that the time difference (Δ t =3.2 ns) between the early and late bins is longer than the width of the laser pulse (4 ps) and coherence time of the biexciton (211 ps) and exciton (119 ps) photons. These laser pulse pairs excite the quantum dot biexciton state through the resonant two-photon excitation process shown in Fig. 1a . Details of the excitation process and experimental set-up can be found in ref. 26 . The schematic of time-bin entanglement generation from a quantum dot and its spectrum are shown in Fig. 1c,b , respectively. The relative phase between the pump pulses creating two-photon excitations is given by φ P = E XX Δ t / ℏ , where E XX is the energy of the biexciton photon. Resonant excitation is crucial as it coherently transfers the phase of the pump pulses and thus the coherence created by the pump interferometer to the biexciton state. The coherence of the excitation process was proved in our previous work [26] , through coherent manipulation experiments demonstrating Ramsey interference. In contrast, other, non-resonant excitation techniques involve phonon transitions, which leak the creation time of the biexciton to the environment [27] , thereby degrading the coherence. At sufficiently low excitation power the biexciton state is created either by the early or by the late pulse, followed by the emission of a biexciton–exciton photon cascade. 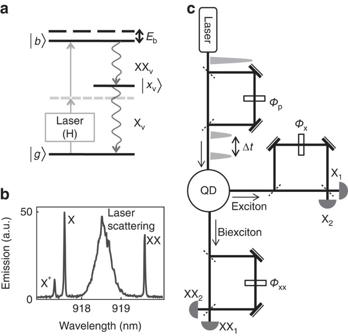Figure 1: Schematic of time-bin entanglement generation and analysis. (a) Energy-level scheme for resonant two-photon excitation of a biexciton (|b›) from the ground state (|g›). The H-polarized pump laser populates the biexciton state resonantly through a virtual level (dashed grey line). Following the excitation, a V-polarized biexciton (XXV) exciton (XV) photon cascade is generated through the intermediate exciton state (|xV›). Exciton and biexciton photons are detuned from the excitation laser due to the biexciton binding energyEb. (b) Quantum dot emission spectrum. (c) Scheme to generate and analyse time-bin entangled photons. Outputs of analysing interferometers, X1, X2, XX1and XX2, are fibre coupled to avalanche photon diodes (APD). Here,φP,φXandφXXare the phases in the pump and analysing interferometers, respectively, and Δtis the time difference between the early and late time bins. The emitted photons are in the time-bin entangled state Figure 1: Schematic of time-bin entanglement generation and analysis. ( a ) Energy-level scheme for resonant two-photon excitation of a biexciton (| b ›) from the ground state (| g ›). The H-polarized pump laser populates the biexciton state resonantly through a virtual level (dashed grey line). Following the excitation, a V-polarized biexciton (XX V ) exciton (X V ) photon cascade is generated through the intermediate exciton state (| x V ›). Exciton and biexciton photons are detuned from the excitation laser due to the biexciton binding energy E b . ( b ) Quantum dot emission spectrum. ( c ) Scheme to generate and analyse time-bin entangled photons. Outputs of analysing interferometers, X 1 , X 2 , XX 1 and XX 2 , are fibre coupled to avalanche photon diodes (APD). Here, φ P , φ X and φ XX are the phases in the pump and analysing interferometers, respectively, and Δ t is the time difference between the early and late time bins. Full size image where the photon pairs are in a coherent superposition of being emitted in the early or late time bin. The subscripts X and XX refer to the exciton and biexciton recombination photon, respectively. We analyse the entanglement of the emitted photons in a time-bin-interference experiment [11] as shown in Fig. 1c . The exciton and biexciton photons are fed into two separate analysing interferometers that have delays equal to the pump interferometer. Finally, we record the coincidences between the outputs of the analysing exciton and biexciton interferometers. Photon pairs produced by the early pulse and taking the long path in the analysing interferometers are indistinguishable from photon pairs produced by the late pulse and taking the short path. Thus, the probability amplitudes of the two possible indistinguishable events interfere. This interference results in a sinusoidal change of the coincidence rates while the phase of one of the interferometers is varied. The relationship between coincidence counts and interferometer phase can be approximated [28] by with i , j taken as +1(−1) for the XX and X outputs 1(2), respectively. Here, φ X(XX) is the phase of the exciton (biexciton) analysing interferometer. The visibility ( V ) of the interference is connected to the quality of the time-bin entanglement and it is ideally equal to unity. In order to achieve maximum visibility the phase ( φ XX + φ X − φ P ) has to be stable during the experiment. This can be accomplished by active stabilization of all three interferometers with respect to a phase-stable laser. In our experiment, the phase stability is achieved by realizing the pump and analysing interferometers in three different spatial modes of a single bulk interferometer as shown in Fig. 2 . We take advantage of the phase relation, such that the relative phase always remains the same independent of the drift in the interferometer. The phase of both the analysing interferometers can be set independently with the phase plates PP X and PP XX . 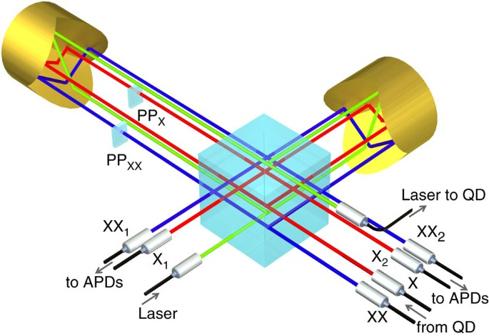Figure 2: One bulk interferometer hosts both the pump and analysing interferometers. The interferometer is built with a 50:50 beam splitter cube and two retro-reflectors. The pump laser and the single photon pairs are in separate spatial modes. In- and out-coupling of photons in the interferometer is made via single-mode fibres. The phases of the biexciton and exciton analysing interferometers are controlled with phase plates, PPXXand PPX. Figure 2: One bulk interferometer hosts both the pump and analysing interferometers. The interferometer is built with a 50:50 beam splitter cube and two retro-reflectors. The pump laser and the single photon pairs are in separate spatial modes. In- and out-coupling of photons in the interferometer is made via single-mode fibres. The phases of the biexciton and exciton analysing interferometers are controlled with phase plates, PP XX and PP X . Full size image Detection in post-selection In order to extract the single events and coincidences between the photons at the outputs of the two analysing interferometers we record the arrival times of the photons with respect to the pump pulse. The triggering to the laser pulse is essential because it allows us to separate distinguishable from indistinguishable events. For example, Fig. 3a shows the recorded single events for the output X 1 . The photons created by the early (late) pulse and travelling the short (long) path form the first (third) peak. The second peak is formed by photons created by the early excitation taking the long path and the photons created by the late excitation taking the short path. For our analysis we post-select only the photons arriving within a window of 1.28 ns in each of the peaks, shaded with grey in Fig. 3a . From the post-selected events we extract coincidences between the outputs of the two analysing interferometers. The resulting histogram has five peaks (see Fig. 4 ). The first (last) peak consists of the pairs created by the early (late) pulse and passing through the short (long) paths of the analysing interferometers. Also, the second and the fourth peaks represent distinguishable events, where the biexciton and exciton photons have travelled along opposite interferometer arms. Thus the second (fourth) peak exclusively shows coincidences created by the early (late) pulse. The third peak shows the indistinguishable events that interfere and exhibit entanglement. 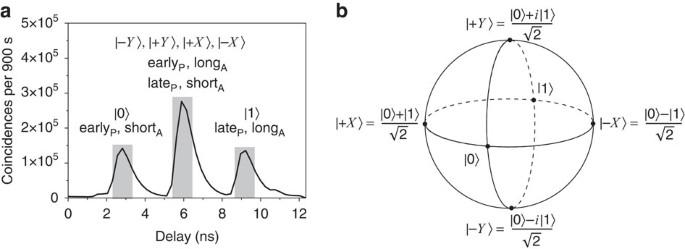Figure 3: Time-bin qubit and Bloch sphere representation. (a) Arrival time of the exciton photons recorded with respected to the pump pulse. The grey-shaded regions are the 1.28 ns windows taken for extracting the triple coincidences (laser–biexciton–exciton). The side peaks are the projections onto the time-basis states |0› and |1›. The middle peak is the projection onto the energy bases |±X› and |±Y› for the phase settingsφX=0 andπ/2, respectively. Here, subscript A stands for the analysing and P for the pump interferometer. (b) The time-bin qubit states are represented on a Bloch sphere. Figure 3: Time-bin qubit and Bloch sphere representation. ( a ) Arrival time of the exciton photons recorded with respected to the pump pulse. The grey-shaded regions are the 1.28 ns windows taken for extracting the triple coincidences (laser–biexciton–exciton). The side peaks are the projections onto the time-basis states | 0 › and | 1 ›. The middle peak is the projection onto the energy bases |± X › and |± Y › for the phase settings φ X =0 and π /2, respectively. Here, subscript A stands for the analysing and P for the pump interferometer. ( b ) The time-bin qubit states are represented on a Bloch sphere. 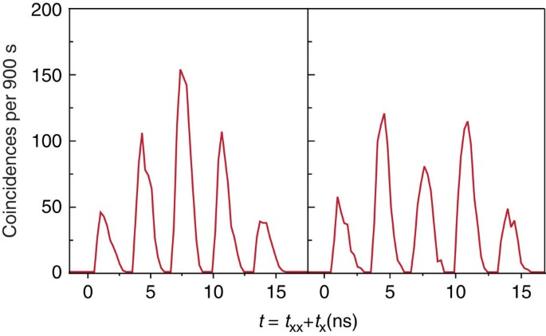Figure 4: Coincidences between biexciton and exciton outputs of the analysing interferometers. The coincidences are triggered on the laser-pulse arrival. The coincidences were recorded for phase settings: (a)φXX+φX=0 and (b)φXX+φX=π. The arrival time is represented as the sumtXX+tX, wheretXX(X)is the arrival time of the biexciton (exciton) recombination photon with respect to the laser trigger. Full size image Figure 4: Coincidences between biexciton and exciton outputs of the analysing interferometers. The coincidences are triggered on the laser-pulse arrival. The coincidences were recorded for phase settings: ( a ) φ XX + φ X =0 and ( b ) φ XX + φ X = π . The arrival time is represented as the sum t XX + t X , where t XX(X) is the arrival time of the biexciton (exciton) recombination photon with respect to the laser trigger. Full size image Tomography measurements We quantify the time-bin entanglement of the emitted photon pairs by measuring their quantum state through quantum state tomography [29] . With this method we reconstruct the density matrix of the generated time-bin entangled photons. We record coincidence events for different projections of the individual qubits (exciton and biexciton photons) to the states |0›, |1›, |+ X › and |+ Y › (represented on the Bloch sphere shown in Fig. 3b ). Projections onto the states | X › and | Y › (energy basis) are achieved by setting the phase in the analysing interferometer to 0 and , respectively. It takes four measurements (see Methods) to obtain all 16 projections of the entangled two-qubit state that are required for the tomographic state reconstruction [29] . The analysing interferometers phase settings for these four measurements are . The real and imaginary parts of the reconstructed density matrix are shown in Fig. 5 , from which we obtain a fidelity of 0.69(3) with respect to the |Φ + › state, a tangle of 0.17(5) and a concurrence of 0.41(6). In addition, the visibilities in three orthogonal bases 0/1, + X /− X and + Y /− Y were measured to be 78.94(2)%, 41.40(3)% and 37.79(3)%, respectively. The raw counts used to reconstruct the density matrix are given in Supplementary Table 1 . 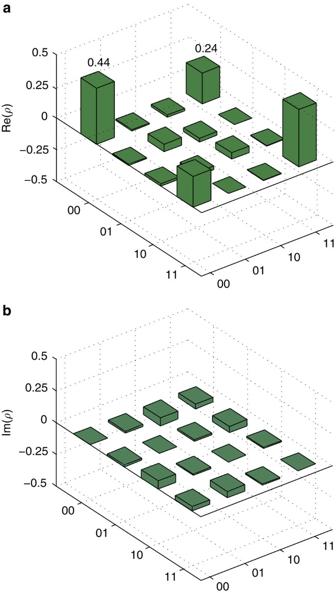Figure 5: Reconstructed density matrixρplotted as a bar chart. (a) Real part. (b) Imaginary part. The reduced value of 0.44 for the 00 (early-early) and 11 (late–late) populations is a consequence of the double excitations that appear as 01 (early–late) and 10 (late–early) populations. The reduced value of the off-diagonal elements (coherences) of about 0.24 comes from the lack of finite coherence of the excitation and emission processes in the quantum dot. Figure 5: Reconstructed density matrix ρ plotted as a bar chart. ( a ) Real part. ( b ) Imaginary part. The reduced value of 0.44 for the 00 (early-early) and 11 (late–late) populations is a consequence of the double excitations that appear as 01 (early–late) and 10 (late–early) populations. The reduced value of the off-diagonal elements (coherences) of about 0.24 comes from the lack of finite coherence of the excitation and emission processes in the quantum dot. Full size image The imperfect interference visibility and hence the reduced fidelity and concurrence of the entangled state can mainly be attributed to double excitation and environment-induced dephasing. Ideally, we expect pairs to be produced in only one of the two pulses. Nevertheless, there is a finite probability that both early and late pulse generate a photon pair. For this first realization of time-bin entanglement we chose a relatively high excitation power as a compromise between the quality of the entanglement and count rate. For this power we calculate from our data a 12.4% contribution of such events. The coincidences between these double excitations form an incoherent background, hence reducing the visibilities in all three orthogonal bases. For example, if we reduced the excitation pulse power by 75% we estimate visibilities of 95.11(3)%, 48.47(3)% and 51.34(3)%, for 0/1, + X /− X and + Y /− Y bases, respectively. Correspondingly we would then obtain 0.48(6) for the tangle, 0.61(6) for the concurrence and 0.79(4) for the fidelity (for details see Supplementary Note 1 ). Beyond double excitations some decoherence of the entangled state originates from the pure dephasing of excitons and biexcitons in the solid-state environment due to phonon interactions and spectral diffusion. These interactions leak information about the creation time of the biexciton [27] and energy fluctuations of the excitons reduce the visibility of two-photon interference. The dephasing in the quantum dot used for the experiment is characterized with lifetime (biexciton: 405 ps, exciton: 771 ps) and coherence length (biexciton: 211 ps, exciton: 119 ps) measurements, which are far from the ideal transform limited condition. Time-bin entanglement measures the mutual coherence between the emission of the early and the late cascade, not the coherence between the individual photons. Therefore we cannot directly use these numbers to calculate the required mutual coherence without a full quantum optical model of the quantum dot and its environment. We generate time-bin entangled photons from a quantum dot using the biexciton–exciton cascade. As far as we know this is the first realization of energy-time entanglement from a single quantum emitter of any type. This was made possible by our method of coherent excitation of the biexciton [26] . Reconstructing the density matrix through quantum state tomography unambiguously confirms the entanglement of the generated photon pairs. At the same time, our source is distinguished from spontaneous parametric down-conversion sources by its sub-Poissonian photon statistics. Because our scheme is not affected by fine-structure splitting it can be applied to a much larger variety of quantum dots than polarization entanglement and it also directly provides the most robust kind of entanglement. Higher extraction efficiencies, which can be achieved with quantum dots in coupled pillar microcavities [19] , would immediately improve the entanglement of our source in two ways: (1) one would be able to measure at lower excitation power for the same count rate, thus reducing the unwanted double excitations, and (2) the Purcell enhancement of the microcavity would improve the indistinguishability [30] of the emitted photons and in turn the two-photon interference. In the long run, to achieve scalability of the source we will need to eliminate the double excitations that reduce the entanglement by identifying a metastable state [24] , [25] that can serve as an initialization state. We expect that such an initialization state will also reduce the dephasing during the coherent excitation process and therefore allow us to reach levels of entanglement achievable by parametric down-conversion ( Supplementary Tables 2 and 3 ). A measurement of the arrival time of a photon at the output of the analysing interferometer with respect to the excitation laser gives rise to the three peaks shown in Fig. 3a . Here, the first and the last peak carry the information on classical correlations (between |0› and |1›) and the middle peak shows quantum correlations. For example, |+ Y , 0› is a projection where the biexciton photon is projected onto the energy basis and the exciton is projected onto the time basis. The joined projections onto the time basis (|0, 0›, |0, 1›, |1, 0›, |1, 1›) are obtained as coincidence events in respective combination of the time intervals measured between the outputs of the analysing interferometers for biexciton and exciton. Projections onto the energy bases (| Y ›, | X ›) are obtained from respective specific phase settings by extracting coincidence events in the time of arrival of the middle peak for the exciton and biexciton signals. Projections with energy and time bases combinations (|0, + Y ›, |+ Y , 0›, |+ Y , 1›, |1, + Y ›, |0, + X ›, |+ X , 0›, |1, + X ›, |+ X , 1›) are collected from coincidence events in the interval of arrival of the respective middle and side peaks. In order to obtain the measurement errors we performed a 100-run Monte Carlo simulation of the data with a Poissonian noise model applied to the measured values. The single count rate in the measurements was 4k counts for both exciton and biexciton, collected and detected in a single-mode fibre. The wavelength of the entangled photons is around 920 nm ( Fig. 1b ). The time resolution of the avalanche photo detector is 200 ps and the quantum efficiency is 20%. We estimate the rate of entangled photon pairs to be 0.6 counts s −1 . How to cite this article: Jayakumar, H. et al . Time-bin entangled photons from a quantum dot. Nat. Commun. 5:4251 doi: 10.1038/ncomms5251 (2014).